Speed control for neuronal migration in the postnatal brain by Gmip-mediated local inactivation of RhoA Throughout life, new neurons generated in the ventricular–subventricular zone take the long journey to the olfactory bulb. The intracellular mechanisms that precisely control the neurons’ migration speed, enabling their well-organized movement, remain unclear. Rho signalling is known to affect the morphology and movement of various cell types, including neurons. Here we identify Gem-interacting protein (Gmip), a RhoA-specific GTPase-activating protein, as a key factor in saltatory neuronal migration. RhoA is activated at the proximal leading process of migrating neurons, where Gmip is also localized and negatively regulates RhoA. Gmip controls the saltatory movement of neurons that regulate their migration speed and ‘stop’ positions in the olfactory bulb, thereby altering the neural circuitry. This study demonstrates that Gmip serves as a brake for the RhoA-mediated movement of neuronal somata, and highlights the significance of speed control in the well-organized neuronal migration and the maintenance of neuronal circuits in the postnatal brain. Neuronal migration is crucial not only for embryonic development but also in the postnatal and adult brain [1] , [2] , [3] , [4] . For the normal development and maintenance of the brain, neurons must migrate at the proper speed along their path and stop upon reaching their destination. Normally, the speed of neuronal migration is not constant, it can be affected by brain development and by the microenvironments surrounding neurons [5] . To control speed tightly, both acceleration and braking systems may be needed. Decreased expression of negative regulators such as srGAP and Cullin-5 (refs 6 , 7 , 8 ) in embryos has been reported to cause cortical neurons to migrate radially at high speed and to fail to stop at the appropriate location. Although the mechanisms that negatively regulate neuronal movement are poorly understood, such an inhibitory system should be particularly important for new neurons that navigate over long distances, through an intricate environment of established tissues, as occurs in the postnatal and adult brain. One of the most complex and difficult migrations undertaken by new neurons is between the ventricular wall, where they are born, and the olfactory bulbs (OBs); this migration begins in the embryonic brain and persists throughout adulthood. During this process, new neurons generated in the ventricular–subventricular zone (V-SVZ) of the lateral walls of the lateral ventricles migrate over a long distance along a pathway called the rostral migratory stream (RMS) towards the OB [9] , [10] , [11] , [12] , [13] . As they migrate, the neurons move along complex mesh-like routes through astrocyte tunnels by forming elongated cell aggregates called ‘chains’ [14] , [15] , and within the aggregates these neurons also move over and past one another [16] . Once in the OB, the neurons migrate radially to their final position in the appropriate layer, where they differentiate into one of the two types of local olfactory interneurons: granule cells (GCs) or periglomerular cells (PGCs) [10] , [17] . The speed of migration in the RMS is about twice that of the radial glia fiber-guided migration of cortical neurons [18] . Altering the speed of migration in the RMS can affect the fate of newborn OB neurons [19] . Previous studies have shown that this complex neuronal migration is regulated through the orchestrated activities of multiple signals. However, little is known about the inhibitory mechanisms that control the speed of neuronal migration or the mechanisms that determine where each neuron should end its migration. As immature neurons migrate, the soma moves in saltatory increments, executed by the repeated growth of the leading process followed by the rapid advancement of the soma [20] , [21] . Before the soma translocates, the centrosome moves forward forming a transient ‘swelling’ in the proximal leading process; the soma, along with the nucleus, then moves towards the centrosome [20] , [22] , [23] . Thus, the translocation of the soma over some distance, which we call a ‘stride,’ followed by a pause, defines a single saltatory movement. Migration occurs as the result of this cycle being repeated many times. The overall migratory speed of a given neuron could be regulated at the level of these migratory components, that is, stride distance, stride frequency and the length of the pause. The dynamic reorganization of F-actin in the soma and the proximal leading process of migrating neurons have an important role in soma translocation [21] . A recent study suggests that Rho signalling via mDia (mammalian diaphanous homologue) and ROCK/Rho-kinase (Rho-associated protein kinase) regulates F-actin dynamics in these cellular compartments to promote the saltatory movement of the soma of new neurons migrating from the V-SVZ to OB [24] , suggesting that F-actin dynamics and organization through the regulation of Rho signalling is essential for neuronal migration. The activity of Rho family small GTPases is tightly regulated by three groups of proteins: guanine nucleotide exchange factors, GTPase-activating proteins (GAPs) and guanine nucleotide dissociation inhibitors [25] , [26] , [27] . However, neither the spatio-temporal pattern of Rho signalling activity in migrating neurons nor its regulatory mechanisms has been studied. Here, we report a novel regulatory mechanism of RhoA and its function in new neurons migrating from the V-SVZ towards the OB in the RMS of the postnatal mouse brain. We identified Gem-interacting protein (Gmip), a RhoA-specific GAP (Rho-GAP) [28] , [29] , in a proteomics screen for proteins interacting with Girdin (Girders of actin), an actin-binding protein essential for neuronal migration to the OB [30] . We demonstrate that RhoA is activated at the proximal leading process, where Gmip is also localized and negatively controls RhoA. Gmip was required for the control of the soma’s saltatory movement by which it regulated the neuronal migration speed in the RMS and OB. Gmip also determined the final positions of new GCs in the OB, thereby influencing the neural circuitry. We propose that Gmip and RhoA are major regulators of neuronal migration in the postnatal brain. Identification of Gmip as a Girdin-interacting protein To identify Girdin-interacting proteins, we performed the immunoprecipitation (IP) of Girdin from a postnatal mouse V-SVZ lysate, followed by a liquid chromatography tandem mass spectrometry (LC-MS/MS) shotgun analysis. We obtained 205 candidates for Girdin-interacting proteins, which included cytoskeletal proteins (5%), cytoskeleton-binding proteins (5%), signal-transduction proteins (19%), nucleic acid-binding proteins (51%) and others (20%). In this study, we focused on one of the signal-transduction proteins, Gmip (Gem-interacting protein; Supplementary Fig. 1a ), a Rho-GAP [28] , [29] . We prepared a specific antibody to characterize the Gmip protein. Western blotting detected the endogenous Gmip protein in a V-SVZ tissue lysate ( Fig. 1a and Supplementary Fig. 1b ). To confirm the interaction between Girdin and Gmip, a lysate of P2 rat V-SVZ tissue was subjected to IP with a control IgG or anti-Girdin antibody, followed by western blot analysis with the anti-Gmip antibody. When the endogenous Girdin was immunoprecipitated, Gmip was detected in the immunoprecipitate ( Fig. 1b and Supplementary Fig. 1c ). Reciprocally, when the same lysate was subjected to IP with control IgG or the anti-Gmip antibody, endogenous Girdin was specifically detected in the immunoprecipitate of the anti-Gmip antibody ( Fig. 1c and Supplementary Fig. 1c ). These results suggest that Girdin and Gmip form a complex in the V-SVZ. 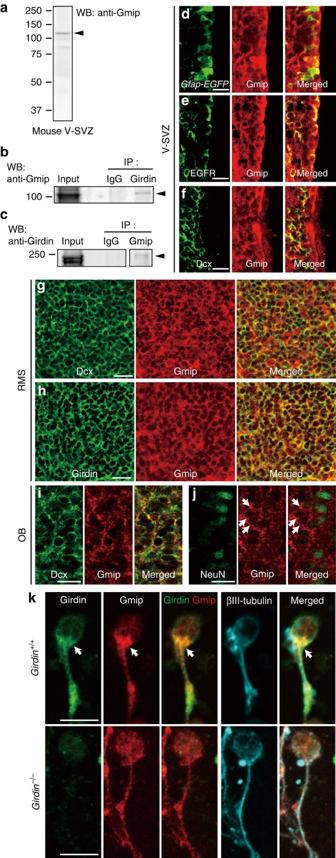Figure 1: Interaction of Gmip with Girdin in postnatal mouse new neurons. (a) Expression of Gmip in the postnatal mouse brain. Lysate of V-SVZ tissue from P5 mice was subjected to immunoblotting using an anti-Gmip antibody. The Gmip protein is indicated by an arrowhead. (b,c) Complex formation between endogenous Gmip and Girdin in brain lysate. The lysate of V-SVZ tissue from P2 rats was subjected to immunoprecipitation (IP) analysis with control IgG or an anti-Girdin antibody, followed by western blot (WB) analysis with anti-Gmip antibody (b). Reciprocally, the same lysate was subjected to IP with control IgG or an anti-Gmip antibody, followed by WB analysis with anti-Girdin antibody (c). Immunoprecipitated proteins are indicated by arrowheads. (d–j) Expression pattern of Gmip in the postnatal V-SVZ, RMS and OB. Coronal sections from P7 mouse brain were stained with anti-Gmip antibody (red) in combination with the indicated antibodies (green). Arrows, Gmip+NeuN- cells (j). (k) Localization of Gmip and Girdin in cultured new neurons from the V-SVZ. New neurons dissociated from the V-SVZ tissue ofGirdin−/−or WT littermate (Girdin+/+) P1–4 mice were fixed at 2 daysin vitro, followed by immunostaining with the indicated antibodies (Gmip: red, Girdin: green and βIII-tubulin: cyan). Arrows, proximal leading process. Scale bars, 20 μm (d–j) and 10 μm (k). For full blots, seeSupplementary Fig. 10. Figure 1: Interaction of Gmip with Girdin in postnatal mouse new neurons. ( a ) Expression of Gmip in the postnatal mouse brain. Lysate of V-SVZ tissue from P5 mice was subjected to immunoblotting using an anti-Gmip antibody. The Gmip protein is indicated by an arrowhead. ( b , c ) Complex formation between endogenous Gmip and Girdin in brain lysate. The lysate of V-SVZ tissue from P2 rats was subjected to immunoprecipitation (IP) analysis with control IgG or an anti-Girdin antibody, followed by western blot (WB) analysis with anti-Gmip antibody ( b ). Reciprocally, the same lysate was subjected to IP with control IgG or an anti-Gmip antibody, followed by WB analysis with anti-Girdin antibody ( c ). Immunoprecipitated proteins are indicated by arrowheads. ( d – j ) Expression pattern of Gmip in the postnatal V-SVZ, RMS and OB. Coronal sections from P7 mouse brain were stained with anti-Gmip antibody (red) in combination with the indicated antibodies (green). Arrows, Gmip+NeuN- cells ( j ). ( k ) Localization of Gmip and Girdin in cultured new neurons from the V-SVZ. New neurons dissociated from the V-SVZ tissue of Girdin −/− or WT littermate ( Girdin +/+ ) P1–4 mice were fixed at 2 days in vitro , followed by immunostaining with the indicated antibodies (Gmip: red, Girdin: green and βIII-tubulin: cyan). Arrows, proximal leading process. Scale bars, 20 μm ( d – j ) and 10 μm ( k ). For full blots, see Supplementary Fig. 10 . Full size image To determine Gmip’s expression pattern, we performed immunohistochemistry. The specificity of the anti-Gmip antibody was confirmed by an antibody absorption experiment ( Supplementary Fig. 1d ). To identify the Gmip-expressing cell types in the V-SVZ, we stained postnatal mouse brain sections with the anti-Gmip antibody in combination with markers for neural stem cells, transit-amplifying cells and new neurons. Using Gfap-EGFP mice, in which green fluorescent protein (GFP) is expressed under the control of the Gfap gene promoter, we found that the majority of the GFP+ V-SVZ astrocytes expressed Gmip (67.5±3.5%, 515 cells from three mice, data represent mean±s.e.m. ; Fig. 1d ). In addition, almost all of the epidermal growth factor receptor+ (EGFR+) activated neural stem/transit-amplifying cells, and doublecortin+ (Dcx+) new neurons expressed Gmip (EGFR+ neural stem/transit-amplifying cells, 95.2±1.3%, 412 cells from three mice; Dcx+ new neurons, 99.4±0.4%, 1,191 cells from three mice, data represent mean±s.e.m. ; Fig. 1e,f ). In the RMS, Dcx+ new neurons expressed both Girdin and Gmip ( Fig. 1g,h ). In the OB, the Gmip expression was maintained in the Dcx+ new neurons ( Fig. 1i ) but it was decreased in the NeuN+ mature GCs in the GC layer (GCL; NeuN+ mature GCs, 15.3±2.0%, 879 cells from three mice, data represent mean±s.e.m. ; Fig. 1j ). Gmip expression was also observed in the mature neurons in the postnatal telencephalon ( Supplementary Fig. 1e ). To observe the subcellular localization of Gmip, new neurons dissociated from postnatal mouse V-SVZ tissue were double stained for Gmip and Girdin. In wild-type (WT) neurons, Gmip and Girdin signals were observed in the whole cytoplasm and were co-accumulated in the proximal leading process at higher levels ( Fig. 1k ; Girdin +/+ ). Interestingly, this accumulation of Gmip was not observed in new neurons from Girdin-deficient neurons ( Fig. 1k ; Girdin −/− ). Instead, Gmip was evenly dispersed throughout the cytoplasm of these neurons, suggesting that Gmip’s proper localization in new neurons is dependent on Girdin. To observe the subcellular localization of Gmip in live migrating neurons, we performed time-lapse imaging of cultured EGFP- or EGFP-Gmip-expressing WT neurons in three-dimensional Matrigel culture. While EGFP was evenly distributed throughout the whole cytoplasm of neurons, EGFP-Gmip was accumulated in the proximal leading process ( Supplementary Fig. 2 ), similar to the localization of endogenous Gmip protein observed in the fixed cultured neurons ( Fig. 1k ). Thus, we identified Gmip as a Rho-GAP protein that colocalizes with Girdin in the proximal leading process of new neurons derived from the V-SVZ in the postnatal brain. Gmip controls the migration of newborn neurons towards the OB To study the role of Gmip in the migration of new neurons ( Fig. 2 ), we first examined the effects of Gmip overexpression. Biochemical assays using full-length Gmip confirmed that Gmip could downregulate RhoA activity ( Fig. 2b,c ; ref. 28 ). We also found that two GAP domain-deleted mutants (GmipΔGAP&cysteine-rich region (CRR) and GmipΔGAP) did not suppress the RhoA activity ( Fig. 2b,c ), suggesting that Gmip’s GAP domain is required for its downregulation of RhoA activity. Control-, Gmip- or GmipΔGAP-expressing plasmids were introduced into the lateral ventricles of P1 mice, and transduced into neural cells by electroporation. Six days post electroporation (6 d.p.e. ), at P7, we counted the labelled cells in the RMS and OB in sagittal brain sections immunostained for GFP ( Fig. 2a ). The percentage of labelled cells that reached the OB was significantly decreased by the overexpression of Gmip but not of GmipΔGAP compared with the control group ( Fig. 2d–g and Supplementary Fig. 3 ). These results suggest that the excessive GAP activity of Gmip disturbed the rostral migration of new neurons into the OB. 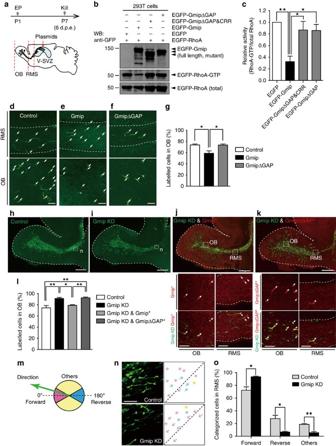Figure 2: Function of Gmip in the migration of new neurons. (a) Experimental scheme. (b,c) Regulation of RhoA activity by the GAP domain of Gmip. The blot intensities (b) were quantified, and the relative RhoA activity was calculated as the ratio of RhoA-GTP/total RhoA (c, three independent experiments). *P<0.05, **P<0.01, one-way ANOVA. (d–f) Effect of Gmip overexpression on the distribution of new neurons. High-magnification images of the boxed areas inSupplementary Fig. 3(white-dashed lines) are shown (d–f). Arrows, labelled cells; asterisks, artifacts. (g) Percentage of labelled cells in the OB (control,n=4 mice (7,457 cells); Gmip,n=5 mice (2,302 cells); GmipΔGAP,n=4 mice (2,324 cells)). *P<0.05, one-way ANOVA. (h–k) Effect of Gmip KD on the distribution of new neurons. Low-magnification images of sagittal brain sections at 6 d.p.e. with control, Gmip KD, Gmip KD & Gmip*, and Gmip KD & GmipΔGAP* vectors are shown (h–k). High-magnification images (j,k) of the OB or RMS regions indicated by squares (white-dashed lines) are also shown. Arrows, labelled cells (KD: green, Gmip* or GmipΔGAP*: red). (l) Percentage of labelled cells in the OB (control,n=3 mice (8,512 cells); Gmip KD,n=3 mice (10,978 cells); Gmip KD & Gmip*,n=4 mice (1,800 cells); Gmip KD & GmipΔGAP*,n=4 mice (2,765 cells)). *P<0.05, **P<0.01, one-way ANOVA. (m–o) Effect of Gmip KD on the direction of new neurons. (m) Mapping of the direction of new neurons. Labelled new neurons were classified into forward, reverse and others. (n) High-magnification images of the RMS regions indicated by squares inh,iand schematic representation of the direction of individual new neurons. The black dashed line represents the orientation towards the OB in the anterior RMS. The pink, blue and yellow arrows correspond to forward, reverse and others, respectively, as indicated inm. (o) Percentage of cells categorized according to direction in the RMS (control,n=3 mice (89 cells); Gmip KD,n=3 mice (93 cells)). *P<0.05, **P<0.01,t-test. Data represent mean±s.e.m. Scale bars, 500 μm (low-magnification pictures inh–k); 50 μm (d–f, high-magnification pictures inj,k,n). EP, electroporation; WB, western blot. For full blot, seeSupplementary Fig. 10. Figure 2: Function of Gmip in the migration of new neurons. ( a ) Experimental scheme. ( b , c ) Regulation of RhoA activity by the GAP domain of Gmip. The blot intensities ( b ) were quantified, and the relative RhoA activity was calculated as the ratio of RhoA-GTP/total RhoA ( c , three independent experiments). * P <0.05, ** P <0.01, one-way ANOVA. ( d – f ) Effect of Gmip overexpression on the distribution of new neurons. High-magnification images of the boxed areas in Supplementary Fig. 3 (white-dashed lines) are shown ( d – f ). Arrows, labelled cells; asterisks, artifacts. ( g ) Percentage of labelled cells in the OB (control, n =4 mice (7,457 cells); Gmip, n =5 mice (2,302 cells); GmipΔGAP, n =4 mice (2,324 cells)). * P <0.05, one-way ANOVA. ( h – k ) Effect of Gmip KD on the distribution of new neurons. Low-magnification images of sagittal brain sections at 6 d.p.e. with control, Gmip KD, Gmip KD & Gmip*, and Gmip KD & GmipΔGAP* vectors are shown ( h – k ). High-magnification images ( j , k ) of the OB or RMS regions indicated by squares (white-dashed lines) are also shown. Arrows, labelled cells (KD: green, Gmip* or GmipΔGAP*: red). ( l ) Percentage of labelled cells in the OB (control, n =3 mice (8,512 cells); Gmip KD, n =3 mice (10,978 cells); Gmip KD & Gmip*, n =4 mice (1,800 cells); Gmip KD & GmipΔGAP*, n =4 mice (2,765 cells)). * P <0.05, ** P <0.01, one-way ANOVA. ( m – o ) Effect of Gmip KD on the direction of new neurons. ( m ) Mapping of the direction of new neurons. Labelled new neurons were classified into forward, reverse and others. ( n ) High-magnification images of the RMS regions indicated by squares in h , i and schematic representation of the direction of individual new neurons. The black dashed line represents the orientation towards the OB in the anterior RMS. The pink, blue and yellow arrows correspond to forward, reverse and others, respectively, as indicated in m . ( o ) Percentage of cells categorized according to direction in the RMS (control, n =3 mice (89 cells); Gmip KD, n =3 mice (93 cells)). * P <0.05, ** P <0.01, t -test. Data represent mean±s.e.m. Scale bars, 500 μm (low-magnification pictures in h – k ); 50 μm ( d – f , high-magnification pictures in j , k , n ). EP, electroporation; WB, western blot. For full blot, see Supplementary Fig. 10 . Full size image Next, we examined the effects of Gmip knockdown (KD) by vector-based RNA interference (RNAi) on newborn neurons. We constructed plasmids containing KD target sequences for Gmip or lacZ (as a negative control), together with a cDNA encoding Emerald green fluorescent protein (EmGFP). We confirmed that the Gmip KD vector efficiently decreased the expression of exogenous Gmip in vitro by western blotting analyses ( Supplementary Fig. 4 ). To study the effects of Gmip KD on neuronal migration, we introduced these plasmids into the lateral ventricles of P1 mice and quantified the number of GFP+ cells in the RMS-OB route at P7 (6 d.p.e.). In contrast to the results of overexpressing Gmip, the percentage of Gmip KD cells in the OB was significantly increased compared with the control ( Fig. 2h,i,l ). This KD phenotype was rescued by coexpressing KD-resistant Gmip (Gmip*) but not GmipΔGAP* ( Fig. 2j–l ). We also found that neither the overexpression nor the KD of Gmip affected the cell proliferation, neuronal specification or cell survival in the V-SVZ and RMS ( Supplementary Fig. 5 ). Taken together, these results suggest that Gmip’s function as a brake depends on its regulatory effect on RhoA activity in the migrating neurons in the RMS. We also studied the effects of Gmip KD on the migratory direction of new neurons in the RMS. For this purpose, we classified the labelled cells in the RMS according to the orientation of the longest leading process as ‘forward’ (towards the OB), ‘reverse’ (towards the V-SVZ) or ‘others’, and quantified the number of cells in each group (see Methods section for details; Fig. 2m–o ). Gmip KD resulted in a significantly increased percentage of categorized cells in the forward group, and a significant decrease in the reverse and others’ groups ( Fig. 2o ). Taken together, these results suggest that Gmip KD promotes the rostral migration of new neurons towards the OB. Gmip regulates the saltatory neuronal movement To clarify the mechanisms by which the Gmip KD promoted the migration of new neurons towards the OB, we next performed live imaging of the control or Gmip KD neurons migrating in cultured brain slices at 3 d.p.e. ( Fig. 3a,b and Supplementary Movie 1 ). To study the migration speed of new neurons, we traced the routes of labelled cell soma that moved towards the OB. The average migration speed was calculated by tracing the total migration route of each neuron over the entire observation period. We found that Gmip KD neurons migrated significantly faster than the control cells ( Fig. 3b,c ). Consistent with this result, we found that Gmip-overexpressing neurons migrated significantly more slowly than control cells (control, 67.7±3.6 μm h −1 , n =20 cells from three mice; Gmip, 32.3±4.7 μm h −1 , n =35 cells from three mice, P <0.001, t -test, data represent mean±s.e.m. ), suggesting that Gmip controls the speed of neuronal migration. 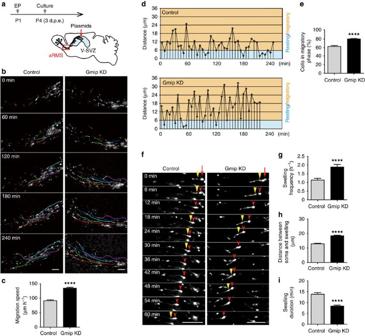Figure 3: Effect of Gmip KD on the speed and movement pattern of new neurons. (a) Experimental scheme. The migration of GFP+ new neurons at 3 d.p.e. with control or Gmip KD vector in the anterior RMS (aRMS, red square) was recorded by time-lapse imaging. (b) Time-lapse sequence of labelled cells migrating in the anterior RMS of brain slices. Five cells in each slice are labelled in the 0-min panel, and their tracks over time are indicated by lines of the same colour (see alsoSupplementary Movie 1). (c) Average migration speed of labelled cells (control,n=68 cells; Gmip KD,n=77 cells, 3 mice each). ****P<0.0001,t-test. (d) Temporal change in the motility of the soma in control and Gmip KD neurons. The migration distance every 6 min was plotted. The blue and orange zones in each graph indicate the resting (0–6 μm) and migratory (>6 μm) phases, respectively. (e) Percentage of cells in the migratory phase (control,n=68 cells; Gmip KD,n=77 cells, 3 mice each). ****P<0.0001,t-test. (f) Examples of time-lapse series of labelled cells in slice culture (high magnification). Red arrows indicate the soma position at the beginning of the observation. Yellow and red arrowheads indicate the swelling and soma, respectively. (g) Average frequency of swellings observed per hour (control,n=18 cells; Gmip KD,n=24 cells, 3 mice each). ****P<0.0001,t-test. (h) Distance between the centre of the soma and the swelling (control,n=28 cells; Gmip KD,n=18 cells, 3 mice each). ****P<0.0001,t-test. (i) Average duration of each swelling (control,n=18 cells; Gmip KD,n=24 cells, 3 mice each). ****P<0.0001,t-test. Data represent mean±s.e.m. Scale bars, 100 μm (b,f). EP, electroporation. Figure 3: Effect of Gmip KD on the speed and movement pattern of new neurons. ( a ) Experimental scheme. The migration of GFP+ new neurons at 3 d.p.e. with control or Gmip KD vector in the anterior RMS (aRMS, red square) was recorded by time-lapse imaging. ( b ) Time-lapse sequence of labelled cells migrating in the anterior RMS of brain slices. Five cells in each slice are labelled in the 0-min panel, and their tracks over time are indicated by lines of the same colour (see also Supplementary Movie 1 ). ( c ) Average migration speed of labelled cells (control, n =68 cells; Gmip KD, n =77 cells, 3 mice each). **** P <0.0001, t -test. ( d ) Temporal change in the motility of the soma in control and Gmip KD neurons. The migration distance every 6 min was plotted. The blue and orange zones in each graph indicate the resting (0–6 μm) and migratory (>6 μm) phases, respectively. ( e ) Percentage of cells in the migratory phase (control, n =68 cells; Gmip KD, n =77 cells, 3 mice each). **** P <0.0001, t -test. ( f ) Examples of time-lapse series of labelled cells in slice culture (high magnification). Red arrows indicate the soma position at the beginning of the observation. Yellow and red arrowheads indicate the swelling and soma, respectively. ( g ) Average frequency of swellings observed per hour (control, n =18 cells; Gmip KD, n =24 cells, 3 mice each). **** P <0.0001, t -test. ( h ) Distance between the centre of the soma and the swelling (control, n =28 cells; Gmip KD, n =18 cells, 3 mice each). **** P <0.0001, t -test. ( i ) Average duration of each swelling (control, n =18 cells; Gmip KD, n =24 cells, 3 mice each). **** P <0.0001, t -test. Data represent mean±s.e.m. Scale bars, 100 μm ( b , f ). EP, electroporation. Full size image To further elucidate the mechanisms of the Gmip KD-induced increase in the speed of neuronal migration, we first plotted the changes in the distance of soma migration every 6 min ( Fig. 3d ). We defined cells in the ‘resting phase’ as those in which the soma travelled <6 μm (<1 μm min −1 ), and those in the ‘migratory phase’ as cells that travelled ≥6 μm (≥1 μm min −1 ). For Gmip KD neurons, the number of cells in the migratory phase was significantly greater ( Fig. 3e ), suggesting that Gmip KD prevents neurons from entering a resting phase. In addition, to analyse the morphology and migration speed of Gmip KD neurons in detail, we observed the morphological changes of migrating neurons in cultured slices. As previously reported [20] , [21] , neurons migrating in cultured brain slices of control and Gmip KD mice had a leading process and exhibited the characteristic saltatory movement of the soma ( Fig. 3f ). That is, the extension of the leading process was followed by the transient formation and anterior movement of the swelling (yellow arrowheads in Fig. 3f ) within the proximal leading process, and then translocation of the soma was initiated. To quantify the frequency of the somatic saltatory movement, we used the swelling as a marker for saltatory strides. The swelling in the proximal leading process appeared more frequently in Gmip KD neurons than in controls ( Fig. 3g ), suggesting that the frequency of somatic strides was significantly higher in these cells. We also measured the distance between the centre of soma and the swelling. In the Gmip KD neurons, the average distance between soma and swelling was significantly greater than in controls ( Fig. 3h ), suggesting that the stride distance was longer. Despite the long stride distance, the duration of each swelling was significantly decreased by Gmip KD ( Fig. 3i ). These results suggest that the somatic translocations of Gmip KD neurons occurred over a greater distance and more frequently than those of controls. Taken together, these findings suggest that Gmip KD speeds up the migration of new neurons by increasing the frequency of the somatic saltatory movement by reducing the resting period and increasing the length of each stride. Gmip is involved in the inactivation of RhoA in new neurons Next, we studied the role of a downstream component of Gmip signalling. Gmip has a Rho-GAP activity [28] and regulates cell morphology in cultured fibroblasts by deactivating RhoA. Although several studies suggested that RhoA is crucial for neuronal migration in the embryonic cerebral cortex [31] , [32] , [33] , [34] , [35] , neither the spatio-temporal activation pattern of RhoA signalling in the migrating OB neurons nor its regulatory mechanisms has been demonstrated. To study the expression of RhoA, we immunostained cultured new neurons dissociated from postnatal mouse V-SVZ tissues. RhoA was detected in the cell body and in the leading process (both on the membrane and in the cytoplasm; Supplementary Fig. 6a ). To investigate the role of RhoA in the migration of OB neurons, we introduced an expression vector encoding a dominant-negative (DN) construct of RhoA into the lateral ventricles of P1 mice, followed by electroporation, and quantified the number of labelled cells in the RMS-OB route at P5 (4 d.p.e.). Compared with the control cells, the percentage of labelled cells observed in the OB was significantly decreased by the expression of DN-RhoA ( Supplementary Fig. 6b,c ), indicating that the inhibition of RhoA activation disturbed the migration of new neurons to the OB. To determine whether Gmip regulates RhoA signalling in newborn OB neurons, we measured the RhoA activity in cultured V-SVZ cells co-transfected with a Förster resonance energy transfer (FRET) biosensor and a Gmip KD or control vector. First, we observed the distribution of active RhoA in control neurons as they formed a swelling. The FRET ratio (=intensity of FRET/cyan fluorescent protein (CFP)) in the swelling was significantly higher than in the trailing process, the distal shaft or the tip of the leading process ( Fig. 4a,b and Supplementary Movie 2 ). This analysis also showed that the FRET ratio in the soma and proximal shaft was significantly higher than in the trailing process. These results suggest that RhoA is activated at the proximal region of the leading process. We occasionally observed a higher FRET ratio at the tip of the leading process compared with that at the distal shaft of the leading process, but the increase was not statistically significant ( Supplementary Movie 2 ). 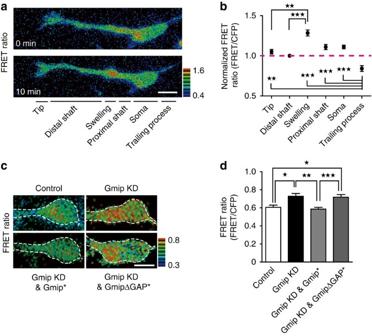Figure 4: Effect of Gmip KD on the RhoA activity in migrating new neurons. (a,b) Analysis of RhoA activity in new neurons. (a) FRET ratio (FRET/CFP) imaging in migrating new neuronsin vitro(see alsoSupplementary Movie 2). The FRET ratio is represented by pseudocolours (see bar at right). (b) Distribution of active RhoA in new neurons. The average normalized FRET ratio of each cell is shown (n=22 cells, six independent experiments). **P<0.01, ***P<0.001, one-way ANOVA. (c,d) Effect of Gmip KD on the RhoA activity in new neurons. Representative images of the analysed cells are shown (c). (d) FRET ratio of the proximal leading process, including the swelling, in the analysed cells (control,n=21 cells; Gmip KD,n=20 cells; Gmip KD & Gmip*,n=46 cells; Gmip KD & GmipΔGAP*,n=28 cells; at least three independent experiments). *P<0.05, **P<0.01, ***P<0.001, one-way ANOVA. Data represent mean±s.e.m. Scale bars, 10 μm (a,c). Figure 4: Effect of Gmip KD on the RhoA activity in migrating new neurons. ( a , b ) Analysis of RhoA activity in new neurons. ( a ) FRET ratio (FRET/CFP) imaging in migrating new neurons in vitro (see also Supplementary Movie 2 ). The FRET ratio is represented by pseudocolours (see bar at right). ( b ) Distribution of active RhoA in new neurons. The average normalized FRET ratio of each cell is shown ( n =22 cells, six independent experiments). ** P <0.01, *** P <0.001, one-way ANOVA. ( c , d ) Effect of Gmip KD on the RhoA activity in new neurons. Representative images of the analysed cells are shown ( c ). ( d ) FRET ratio of the proximal leading process, including the swelling, in the analysed cells (control, n =21 cells; Gmip KD, n =20 cells; Gmip KD & Gmip*, n =46 cells; Gmip KD & GmipΔGAP*, n =28 cells; at least three independent experiments). * P <0.05, ** P <0.01, *** P <0.001, one-way ANOVA. Data represent mean±s.e.m. Scale bars, 10 μm ( a , c ). Full size image Next, we compared the FRET ratio at the proximal leading process, including the swelling, between the control and Gmip KD cells. We found that the FRET ratio was significantly increased by Gmip KD ( Fig. 4c,d ). We next tested the effects of two KD-resistant Gmip mutants (Gmip* and GmipΔGAP*) on the RhoA activity. The RhoA activity at the proximal leading process was significantly decreased by the expression of Gmip* (0.69±0.04, n =30 cells) but not of GmipΔGAP* (0.75±0.04, n =40 cells), compared with control (0.86±0.03, n =64 cells; P <0.01, Gmip; P >0.05, GmipΔGAP (at least three independent experiments, one-way analysis of variance (ANOVA), data represent mean±s.e.m.). Furthermore, the Gmip KD-induced increase in RhoA activity was rescued by the coexpression of Gmip* but not of GmipΔGAP* ( Fig. 4c,d ). Taken together, these results suggest that Gmip’s GAP activity is required for the downregulation of RhoA activity at the proximal leading process in new neurons. Gmip controls the distribution of new neurons in the OB Finally, we studied the effect of Gmip KD on neuronal migration within the OB. We compared the migration speed of control and Gmip KD neurons in each OB layer using time-lapse imaging of cultured brain slices ( Fig. 5a,b and Supplementary Movie 3 ). We found that these neurons gradually slowed during their radial migration in the GCL ( Fig. 5b ). Gmip KD neurons migrated significantly faster than control cells in the deep GCL ( Fig. 5b ), suggesting that the Gmip KD impaired neurons’ deceleration in the OB. 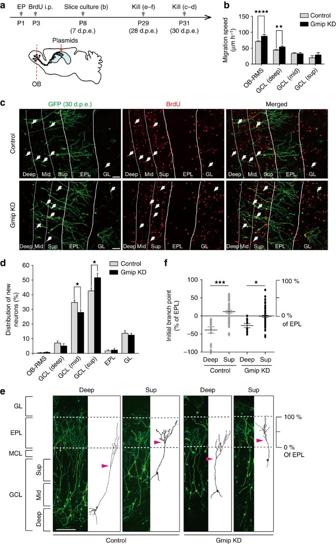Figure 5: Effect of Gmip KD on the migration and distribution of new neurons in the OB. (a) Experimental scheme. (b) Average migration speed of GFP+ cells in each layer of the OB (RMS,n=87 cells (control),n=83 cells (Gmip KD); deep GCL,n=91 cells (control),n=58 cells (Gmip KD); middle GCL,n=36 cells (control),n=15 cells (Gmip KD); superficial GCL,n=3 cells (control),n=9 cells (Gmip KD); from five mice each). **P<0.01, ****P<0.0001,t-test (see alsoSupplementary Movie 3). (c) Distribution of newborn neurons in the OB. Coronal brain sections of the OB at 30 d.p.e. were stained for GFP (green) and BrdU (red). The borders of the GCL, EPL and GL are marked by bold white lines. The GCL was divided into three sublayers (deep, middle (mid) and superficial (sup)), marked by thin white lines. Arrows, GFP+BrdU+ labelled cells. (d) Percentage of labelled new neurons in each layer of the OB (control,n=5 mice (1,167 cells); Gmip KD,n=5 mice (566 cells)). *P<0.05,t-test. (e) Representative examples of control or Gmip KD neurons (left panel, green; right panel, reconstructed images). Red arrowheads indicate the position of the initial branch point of the apical dendrite. (f) Distribution of initial branch points (deep GCs,n=12 cells (control),n=10 cells (Gmip KD); superficial GCs,n=56 cells (control),n=70 cells (Gmip KD); from four mice each). *P<0.05, ***P<0.001, one-way ANOVA. Data represent mean±s.e.m. (b,d). Inf, data represent each point, and the mean±s.e.m. are shown as horizontal bars. Scale bars, 100 μm (c,e). EP, electroporation; i.p., intraperitoneal. Figure 5: Effect of Gmip KD on the migration and distribution of new neurons in the OB. ( a ) Experimental scheme. ( b ) Average migration speed of GFP+ cells in each layer of the OB (RMS, n =87 cells (control), n =83 cells (Gmip KD); deep GCL, n =91 cells (control), n =58 cells (Gmip KD); middle GCL, n =36 cells (control), n =15 cells (Gmip KD); superficial GCL, n =3 cells (control), n =9 cells (Gmip KD); from five mice each). ** P <0.01, **** P <0.0001, t -test (see also Supplementary Movie 3 ). ( c ) Distribution of newborn neurons in the OB. Coronal brain sections of the OB at 30 d.p.e. were stained for GFP (green) and BrdU (red). The borders of the GCL, EPL and GL are marked by bold white lines. The GCL was divided into three sublayers (deep, middle (mid) and superficial (sup)), marked by thin white lines. Arrows, GFP+BrdU+ labelled cells. ( d ) Percentage of labelled new neurons in each layer of the OB (control, n =5 mice (1,167 cells); Gmip KD, n =5 mice (566 cells)). * P <0.05, t -test. ( e ) Representative examples of control or Gmip KD neurons (left panel, green; right panel, reconstructed images). Red arrowheads indicate the position of the initial branch point of the apical dendrite. ( f ) Distribution of initial branch points (deep GCs, n =12 cells (control), n =10 cells (Gmip KD); superficial GCs, n =56 cells (control), n =70 cells (Gmip KD); from four mice each). * P <0.05, *** P <0.001, one-way ANOVA. Data represent mean±s.e.m. ( b , d ). In f , data represent each point, and the mean±s.e.m. are shown as horizontal bars. Scale bars, 100 μm ( c , e ). EP, electroporation; i.p., intraperitoneal. Full size image To study the arrival and final distribution of newborn neurons in the OB, a control or Gmip KD vector was introduced into the lateral ventricles of P1 WT mice, and bromodeoxyuridine (BrdU) was injected at P3. Although new neurons in the Gmip KD group migrated faster than those in the control group ( Figs 2h–l , 3b,c and 5b ), almost all of the GFP+BrdU+ labelled cells eventually reached the OB in both the control and Gmip KD groups by 14 days after BrdU injection (control: 98.1±0.9%, n =416 cells, four mice; Gmip KD: 98.6±1.4%, n =467 cells, four mice; P >0.05, t -test, data represent mean±s.e.m.). Four weeks later (at P31), we quantified the number of labelled cells in each OB layer. Gmip KD increased the percentage of labelled cells in the superficial GCL (superficial GCs) and decreased that in the middle GCL (middle GCs), compared with the control group ( Fig. 5c,d ). The increase in the number of labelled cells in the superficial GCL could be explained by a disturbed migration of PGCs as well as the overmigration of GCs. However, there were no significant differences in the percentage of labelled cells in the external plexiform layer (EPL) and glomerular layer (GL) between the control and Gmip KD groups, suggesting that Gmip KD PGCs could move out of the GCL towards the GL ( Fig. 5c,d ). The change in neuronal distribution in the GCL by Gmip KD was stable and maintained 8 weeks later ( Supplementary Fig. 7 ). There was no significant difference in the proportion of labelled cells that were cleaved caspase-3+ apoptotic cells in any OB layer between the control and Gmip KD groups after reaching the OB ( Supplementary Table 1 ), suggesting that Gmip KD does not affect the survival of new neurons after reaching the OB. Taken together, these results indicate that the Gmip KD induced the overmigration of newly generated neurons to the outer, superficial GCL of the OB. In the control group, the dendritic branches of the superficial GCs ramified predominantly in the superficial EPL, whereas those of the deep GCs were mostly confined to the deep EPL ( Fig. 5e,f ), as previously reported [36] , [37] . To compare the arborizations, we determined the depth of the initial branch point, a surrogate measure of dendritic innervation patterns [37] , and found that the dendrites extending to the superficial EPL by the Gmip KD superficial GCs were similar to those of the control group ( Fig. 5e,f ; for other dendrite measures, see Supplementary Fig. 8 ) [36] , [37] . Thus, the redistributed neurons elaborated dendritic structures that were appropriate for the position of the soma. Taken together, these findings suggest that the Gmip KD impaired the deceleration of new neurons, causing their overmigration in the GCL, and thereby altered their innervation patterns. The present study has demonstrated a new migratory mechanism in which the regulation of RhoA activity controls the speed of new neurons migrating between the V-SVZ and OB in the postnatal brain and the stop positions of these neurons in the OB. RhoA is activated at the proximal leading process, where Gmip, a Rho-GAP, is localized and negatively regulates RhoA. Gmip reduces the average speed of somatic saltatory movements by reducing the stride frequency and distance, and alters the final destinations of new neurons in the OB. Although the spatio-temporal activation of RhoA signalling has been implicated in the migration of various cell types [38] , where and how RhoA activation affects the migration of new neurons has been unclear. We used FRET imaging to determine the RhoA activation sites in migrating neurons, and observed higher activity in the proximal region of the leading process, including the soma and the swelling. When the swelling formed in the proximal leading process, high RhoA activity was observed at the swelling site ( Fig. 4a,b ). During movement cycles, the site containing active RhoA moved with the cells’ morphological change. These results suggest that a periodic change in RhoA activation in the proximal leading process has an important role in migrating neurons. Consistent with this finding, a recent report showed that new V-SVZ neurons deficient in mDia, a Rho-regulated actin nucleator, exhibit impaired migration towards the OB [24] , which is a phenocopy of the DN-RhoA cells described here ( Supplementary Fig. 6b,c ). These results suggest that the control of local RhoA signalling in the proximal leading process is important for the regulation of neuronal migration in the postnatal brain. Gmip was originally identified as a RhoA-GAP that controls cell morphology and polarity in cultured fibroblasts [28] , [29] . A recent study revealed that Gmip-mediated inactivation of RhoA controls vesicular dynamics and azurophilic granule exocytosis in neutrophils, by regulating actin dynamics [39] . Although its in vivo function in the CNS has been unknown, an intriguing association between genetic variations of the GMIP gene and major depressive disorder was reported [40] . Here we showed that Gmip KD cell autonomously promotes neuronal migration from the V-SVZ to the OB. New neurons accomplish their migration through repetitive cycles of somatic saltatory movement, composed of somatic translocation followed by a pause [20] , [21] , which suggests that the coordination of stride distances and the duration of the pause between movements is involved in the speed-control system. Consistent with this, we found that Gmip KD increased both the frequency of saltatory movements, by shortening the pause duration, and the stride length, both of which led to an increase in the speed of neuronal migration from the V-SVZ to OB. Similar regulatory mechanisms may also affect neuronal migration in other brain regions, such as the Cullin-5-mediated saltatory movement of radially migrating pyramidal neurons [7] , [8] . Thus, our findings suggest that the speed of neuronal migration can be precisely controlled by Gmip-mediated modulation of the stride frequency and length in the saltatory movement of the soma. Previous studies suggest that RhoA signalling regulates various steps of neuronal migration in the postnatal RMS [24] , [41] , [42] , [43] . We demonstrated here that DN-RhoA strongly inhibited neuronal migration in the postnatal RMS ( Supplementary Fig. 6b,c ). Although the conditional knockout of RhoA does not cause visible defects in the neuronal migration towards the embryonic OB, it is possible that RhoA has redundant roles with other Rho GTPases, such as RhoC [44] . Since RhoA has several upstream regulators, it is possible that the spatio-temporal regulation of the local RhoA activity by these upstream factors controls neuronal migration in the RMS. In this study, we found that the Gmip protein was weakly expressed throughout the cytoplasm of migrating neurons, and it was higher in the proximal leading process. The accumulation of Gmip in the proximal leading process was not observed in Girdin-deficient neurons ( Fig. 1k ), suggesting that Girdin controls Gmip’s localization to regulate RhoA signalling in a local manner. These data suggest that the sustained activation of RhoA by Gmip KD in the proximal leading process promotes the somatic saltatory movement and thereby the speed of neuronal migration. Since actomyosin-based contraction in the proximal leading process promotes both centrosomal and somatic translocation [21] , the enhancing effects of Gmip KD on somatic saltatory movement are plausibly owing to alterations in RhoA-controlled actomyosin dynamics. In support of this idea, inactivation of the RhoA signal by an mDia deficiency results in the abnormal regulation of the actin cytoskeleton in the proximal leading process, resulting in defective movement of the centrosome and cell soma towards the swelling [24] . Thus, Gmip-mediated regulation of RhoA activity may control the stride distance and frequency of the somatic saltatory movement through cytoskeletal rearrangements, significantly impacting the average speed of the long-distance migration of new neurons in the postnatal RMS ( Supplementary Fig. 9 ). In the RMS, a substantial population of neurons extends their leading process laterally or posteriorly, in addition to the majority of cells that migrate anteriorly. For the long-distance migration in the RMS, not only stride frequency and length, but also directionality may affect the average speed. We found that the percentage of forward-directed migrating neurons in the RMS was significantly increased by Gmip KD. Since the reverse migration of cerebellar GCs is accompanied by the anterior downregulation of RhoA activity [45] , the suppression of RhoA by a Rho-GAP is probably involved in their change in direction. It is possible that the failure to switch-off RhoA activity in Gmip KD cells caused the decreased frequency of turning. Thus, RhoA activity may also affect the directional control of neuronal migration in the RMS, as part of the migratory speed regulation. After reaching the OB, new neurons detach from the RMS and migrate radially to their final positions in the GCL or GL, where they differentiate into GCs or PGCs, respectively [10] , [17] . In the GCL, GCs not only exhibit distinct morphologies and dendritic projection patterns from sub-layer to sub-layer, but also have different synaptic innervations and inhibitory functions for olfactory inputs [36] , [37] . We found that Gmip KD increased the percentage of new GCs distributed to the superficial layers of the GCL owing to the insufficient deceleration of migrating neurons in the OB, although the redistributed cells’ dendritic morphology was similar to that of the naive superficial GCs ( Fig. 5 and Supplementary Fig. 8 ). These data indicate that the regulation of the speed and stopping points of migrating neurons by Gmip affects even the neurons’ innervation pattern, which is reported to be dependent on the timing and location of their birth in the V-SVZ [37] , [46] , [47] . In addition to the lack of significant differences in the dendritic morphology between the Gmip KD and control neurons in each layer of the GCL ( Fig. 5e,f and Supplementary Fig. 8 ), our observation that the Gmip expression progressively decreased after the new neurons stopped in the OB ( Fig. 1j ), when dendrites develop [13] , also suggests that Gmip does not directly regulate dendritic development in the mature GCs in the OB. On the other hand, RhoA has been implicated in the control of dendritic morphogenesis in other neurons [48] , [49] , [50] . Therefore, although Gmip did not affect dendritic development, at least with regard to the initial branching point, branching number or total length of dendrites and branches ( Fig. 5e,f and Supplementary Fig. 8 ), we cannot completely rule out the possibility that the Gmip-mediated local inactivation of RhoA is involved in controlling dendritic development. Taken together, these results highlight the significance of the precisely controlled migration of new neurons in the development and maintenance of the normal neuronal circuitry of the OB. Our results suggest that the periodic inactivation of RhoA by Gmip in migrating neurons controls the speed of migration from the V-SVZ to the OB by regulating the saltatory movement of the soma. Such a speed-control mechanism should be particularly important for the neuronal migration from the postnatal V-SVZ to the OB, which is one of the longest and fastest journeys undertaken by neurons in the brain. Since the migration of V-SVZ neurons towards injured brain tissues is slow and irregular [51] , understanding the mechanisms that control the speed, direction and termination of postnatal neuronal migration may contribute to the development of methodologies that promote neuronal regeneration. Animals Wild-type Institute of Cancer Research mice and Wistar rats were purchased from Japan SLC, Inc. (Shizuoka, Japan). Construction of the Girdin gene-targeting vector and generation of Girdin −/− mice were described previously [52] . Gfap-EGFP mice were obtained from the Mutant Mouse Regional Resource Center (Columbia, MO). All animal experimental procedures complied with national regulations and guidelines were reviewed by the Institutional Laboratory Animal Care and Use Committee, and were approved by the President of Nagoya City University. Antibodies To generate Gmip antibodies, cDNA encoding the Gmip N terminus (amino acids 1–251) or C terminus (amino acids 757–971) was ligated into a pGEX-4T, glutathione S -transferase (GST) fusion expression vector (Pharmacia, Piscataway, NJ). Recombinant GST-Gmip-NT and GST-Gmip-CT proteins were affinity purified using Glutathione Sepharose 4B beads (GE Healthcare, Piscataway, NJ) according to the manufacturer’s instructions and used to immunize rabbits. The specific antibodies were affinity purified from the antisera using recombinant maltose-binding protein (New England Biolabs, Ipswich, MA) fused to the Gmip N terminus or C terminus. To confirm the specificity of the anti-Gmip antibody for immunostaining, we performed an antigen-absorption test. Purified GST or GST-fusion Gmip protein was incubated with Glutathione Sepharose 4B beads for 30 min at 4 °C, and the supernatant was removed. The resulting GST- or GST-Gmip-coated beads were then incubated with the Gmip antibody overnight at 4 °C. After centrifugation at 20,000 g for 1 min at 4 °C, the supernatant was recovered as GST- and GST-Gmip-absorbed Gmip antibodies. Other antibodies used in this study included sheep anti-Girdin polyclonal antibody (1:100, R&D Systems, Minneapolis, MN), rabbit anti-EGFR polyclonal antibody (1:100, Santa Cruz Biotechnology, Santa Cruz, CA), rabbit anti-cleaved caspase-3 antibody (1:200, Cell Signaling Technology, Beverly, MA), goat anti-Dcx polyclonal antibody (1:100, Santa Cruz Biotechnology), rabbit anti-Dcx polyclonal antibody (1:200, Cell Signaling Technology), mouse βIII-tubulin antibody (1:1,000, Sigma, St Louis, MO), rabbit anti-GFP polyclonal antibody (1:1,000, MBL, Nagoya, Japan), rat anti-GFP polyclonal antibody (1:200, Nacalai tesque, Kyoto, Japan), rabbit anti-DsRed antibody (1:1,000, Clontech Laboratories, Inc., Mountain View, CA), mouse anti-β-actin monoclonal antibody (1:500, Roche, Basel, Switzerland), sheep anti-BrdU antibody (1:1,000, Fitzgerald Industries International, Acton, MA), mouse anti-NeuN monoclonal antibody (1:100, Millipore, Billerica, MA), normal sheep IgG, and normal rabbit IgG (10 μg ml −1 , Santa Cruz Biotechnology). The anti-RhoA/C antibody (LULU51, 1:250) was kindly provided by Dr Shigenobu Yonemura, RIKEN Center for Developmental Biology [53] . IP and western blot analysis SVZ tissues and COS7 cells were homogenized in lysis buffer (20 mM Tris–HCl, pH 8.0, 100 mM NaCl, 1 mM EDTA, 10 μg ml −1 leupeptin and 10 μM phenylmethylsulfonyl fluoride (PMSF)). Lysates were briefly sonicated and cleared by centrifugation, followed by IP using the indicated antibodies. For western blot analyses, samples were separated by SDS-polyacrylamide gel electrophoresis. Proteins were transferred to polyvinylidene difluoride (PVDF) membranes, blocked in 0.5% skim milk in Tris Buffered Saline (TBS) containing 0.01% Tween 20, incubated with primary antibodies and detected by horseradish peroxidase-conjugated secondary antibodies (Dako, Glostrup, Denmark) with enhanced luminal-based chemiluminescent western blotting detection reagent (GE Healthcare). Signals were detected and measured with a cooled charge-coupled device camera (LAS3000mini; Fujifilm, Tokyo, Japan). Mass spectrometry The proteins in the immunoprecipitate were digested by trypsin for 16 h at 37 °C after reduction, alkylation, demineralization and concentration. Nanoelectrospray tandem mass analysis was performed using an LTQ Orbitrap XL (Thermo Fisher Scientific, Inc., Waltham, MA) system connected to an HTC-PAL autosampler and a Paradigm MS4 HPLC (Michrom Bioresources, Auburn, CA) with a C18 reversed-phase column and Michrom’s ADVANCE Plug and Play Nano Source (Michrom Bioresources). Reversed-phase chromatography was performed with a linear gradient (0 min, 5% B; 45 min, 100% B) of solvent A (2% acetonitrile with 0.1% trifluoroacetic acid) and solvent B (98% acetonitrile with 0.1% trifluoroacetic acid) at an estimated flow rate of 500 nl min −1 . A precursor ion scan was carried out using a 396–2,000 mass to charge ratio ( m/z ) before MS/MS analysis. Multiple MS/MS spectra were submitted to the programme Mascot (Matrix Science, Inc., Boston, MA) for the MS/MS ion search. Immunohistochemistry Brains were fixed by transcardiac perfusion with 4% paraformaldehyde in 0.1 M phosphate buffer, postfixed overnight in the same fixative, and 60-μm-thick floating coronal or sagittal sections were prepared using a vibratome (VT1200S, Leica, Heidelberg, Germany) as reported previously [15] , [54] . For immunostaining, the sections were incubated for 1 h in blocking solution (10% donkey serum and 0.2% Triton X-100 in PBS), overnight at 4 °C with the primary antibodies, and for 2 h at room temperature with Alexa Fluor-conjugated secondary antibodies (Invitrogen, Carlsbad, CA). Signal amplification was performed with biotinylated secondary antibodies (Jackson Laboratory, West Grove, PA) and the Vectastain Elite ABC kit (Vector Laboratories, Burlingame, CA), and the signals were visualized using the TSA Fluorescence System (PerkinElmer, Waltham, MA). For BrdU staining, the sections were treated with 2 N HCl for 40 min at 60 °C. For double staining using anti-Gmip and EGFR antibodies, sequential immunostaining was performed with AffiniPure Fab Fragment Donkey Anti-Rabbit IgG (H+L) (Jackson ImmunoResearch Laboratories, Inc., West Grove, PA). Nuclei were stained with Hoechst33342 (Sigma). Confocal images were obtained using an LSM5-Pascal or LSM700 laser-scanning microscope system (Carl Zeiss, Jena, Germany). Quantitative analysis To examine the expression pattern of Gmip ( Fig. 1 ), the colocalization of signals in the V-SVZ, RMS and OB was analysed and the double-positive cells in 60-μm-thick coronal sections were counted. To quantify the distribution of GFP+cells in the RMS and OB ( Fig. 2 and Supplementary Fig. 6 ), images of the cells were acquired using a fluorescence microscope, BX51 (Olympus, Tokyo, Japan) and a CCD camera, DP71 (Olympus), and all of the cells in the RMS and OB in 60-μm-thick sagittal sections were counted. To quantify the distribution of GFP+DsRed+ cells in the RMS and OB ( Fig. 2 ), images of the cells were acquired using an LSM700 confocal laser-scanning microscope, and all of the GFP+DsRed+cells in the RMS and OB in 60-μm-thick sagittal sections were counted. To quantify the directionality of migrating neurons ( Fig. 2 ), all of the GFP+ cells whose whole cell morphology could be observed in the RMS were photographed using an LSM5-Pascal or LSM700 confocal microscope, and reconstructions were performed from confocal z-series stacks (20–25 μm) by scanning at 1-μm intervals. To quantify the direction of migrating neurons in the RMS, the angle between the longest leading process and the direction defined as 0° (in the direction of the OB and parallel to the longitudinal arrays of neuron chains) was measured using National Institutes of Health ImageJ. The opposite direction was defined as 180°. GFP+ cells with the longest leading process extending in a direction within a 30° angle on either side of 0° towards the OB were defined as forward-directed cells (described as ‘forward’), those within a 30° angle on either side of 180° were defined as reverse-directed cells (described as ‘reverse’), and those in all other directions were designated as ‘others,’ as previously reported [19] , [54] , [55] . To quantify the number of GFP+BrdU+Dcx+ cells or GFP+BrdU+cleaved caspase-3+ cells in the V-SVZ and RMS ( Supplementary Fig. 5 ), images of the cells were acquired using an LSM700, and all of the triple-positive cells in every sixth 60-μm-thick coronal section were counted. To quantify the distribution of GFP+BrdU+ cells within the OB ( Fig. 5 ), confocal images were obtained using an LSM700, and reconstructions were performed from confocal z-series stacks (30–40 μm) by scanning at 2-μm intervals. The GCL was divided into three layers: the deep, middle and superficial regions on the basis of the nuclear staining pattern. The actual number of GFP+BrdU+ cells in every sixth 60-μm-thick coronal section was counted by the investigator (MM) blind to the group identification of each section, and then the total number of the cells was estimated and the percentage of the cells in each layer was calculated. To assess the dendritic innervation patterns of GFP+ cells within the GCL, we measured the initial branch point of the apical dendrite. The position of the initial branch point in the EPL was calculated as the percentage of the distance from the deep boundary of the EPL to the superficial boundary. The dendritic branching patterns of GFP+cells were reconstructed and quantified using Neurolucida (MBF Biosciences, Williston, VT). Overexpression and RNAi constructs Gmip fragment was obtained from full-length mouse Gmip cDNA (Open Biosystems) by PCR (for primers, see Supplementary Table 2 ). To generate pEGFP-N1-Gmip, Gmip fragment was inserted into pBluescript II between EcoRV sites and replaced it to pEGFP-N1 (Clontech Laboratories, Inc.) between SalI sites. The KD-resistant Gmip (Gmip*) was created by introducing three silent mutations into Gmip at nucleotides 1,424–1,444 (5′-ATGG C GTAGG A AGCCC A TTCA-3′; underline indicates mutations) by PCR. To generate pDsRed-Express1-Gmip* or ptdTomato-N1-Gmip*, the fragment encoding Gmip* was removed from pEGFP-N1-Gmip* between SalI sites and inserted to the corresponding sites of pDsRed-Express1 (Clontech Laboratories, Inc.) or ptdTomato-N1 (Clontech Laboratories, Inc.). The deletion mutants Gmip (GmipΔGAP and GmipΔGAP&CRR) were created by deleting the sequence including GAP or GAP&CRR (nucleotides 1,684–2,190 or 1,192–2,190), respectively, by PCR. The GFP-tagged RhoA N19 expression construct (pEGFP-C1-DN-RhoA) was used as DN-RhoA. For the KD experiments, the targeting sequences of mouse Gmip (Gmip BLOCK-IT miR RNAi Select Mmi58,0340 (5′-ATGGAGTAGGCAGCCCGTTCA-3′), used as Gmip miRNA, Invitrogen) and lacZ (control) were cloned into a modified Block-iT Pol II miR RNAi expression vector containing EmGFP or DsRed-Express (Invitrogen). DNA cassettes containing EmGFP or DsRed-Express and the miRNA sequence were cloned into the modified pCAGGS vector [56] using the Gateway system (Invitrogen). For the validation of KD efficiency, COS7 cells were co-transfected with pEGFP-N1-Gmip and the miRNA expression vector against Gmip (pCAGGS-EmGFP-miR-Gmip miRNA) or lacZ (pCAGGS-EmGFP-milacZ, as a control) using Lipofectamine LTX Plus reagent (Invitrogen). Forty-eight hours after transfection, cell lysates were separated and analysed by SDS-polyacrylamide gel electrophoresis, followed by immunoblotting with the indicated antibodies. All of the plasmids were prepared using Plasmid Maxi Kit (Qiagen, Calencia, CA), and the sequences were confirmed by DNA sequencing. RhoA-GTP pulldown assay HEK293T cells were transfected with EGFP-RhoA together with a construct expressing EGFP (control), EGFP-Gmip, or a GAP domain-deleted EGFP-Gmip mutant (EGFP-GmipΔGAP&CRR or EGFP-GmipΔGAP). Forty-eight hours after transfection, the cells were lysed and subjected to a RhoA-GTP pulldown assay using GST-Rhotekin Rho-binding domain (RBD) peptide (Rho Assay Reagent, Millipore), according to the manufacturer’s instructions. Electroporation and BrdU labelling in vivo Electroporations of P1–2 WT mice were performed as described previously [57] , [58] with some modifications. Briefly, mice were anaesthetized by nitrous oxide and isoflurane and fixed to the platform of a stereotaxic injection apparatus (David Kopf Instruments, Tujunga, CA) by a craniophore. Plasmid solution (1.2 μl of a 2.5–5 μg μl −1 solution) containing 0.01% fast green solution was injected into the lateral ventricles of each mouse, and electronic pulses (70 V, 50 ms, four times) were applied using an electroporator (CUY-21SC; Nepagene, Chiba, Japan) with a forceps-type electrode (CUY650P7). At P3, mice were intraperitoneally injected with BrdU (50 mg kg −1 ) diluted with PBS. Time-lapse analyses of new neurons migrating in brain slices Organotypic brain slices were prepared from P4–9 mice (3–8 days after electroporation with the control or Gmip KD vectors) as reported previously [15] , [55] with modifications. Dissected brains were cut into 300-μm-thick sagittal slices with a vibratome, then cultured on a filter membrane (Millipore) submerged in Neurobasal medium (Invitrogen) supplemented with 10% fetal bovine serum, 2 mM L -glutamine, 2% B-27 (Invitrogen), and 50 U ml −1 penicillin–streptomycin. Before recording, the slices were cultured for 1–3 h in a stage-top chamber at 37 °C in a 5% CO 2 incubation system (Tokai hit, Nagoya, Japan). Time-lapse video recordings were obtained using an inverted light microscope (Axio-Observer, Carl Zeiss) equipped with the Colibri light-emitting diode light system, at low magnification using a × 10 dry objective lens. Every 6 min, images were obtained automatically for 4–8 h. The migration speed and distance between the soma and swelling in the proximal leading process was quantified using National Institutes of Health ImageJ software. V-SVZ cell culture The SVZ was dissected from P1–P4 Girdin knockout and their littermate mice in L-15 medium (Invitrogen) and dissociated with trypsin–EDTA (Invitrogen). The cells were spread onto coverglasses coated with poly- L -lysine (Sigma) and laminin (Invitrogen) at a density of 2.5 × 10 5 cells per point, then cultured in neurobasal medium (Gibco, Big Cabin, OK) containing 10% fetal bovine serum, 50 U ml −1 penicillin–streptomycin (Gibco), 2 mM L -glutamine (Gibco), and 2% B-27 supplement (Gibco). Forty-eight hours after seeding, the cells were fixed with 4% paraformaldehyde. Time-lapse imaging of migrating neurons in Matrigel culture The dissociated V-SVZ cells from P0–P2 WT mice were transfected with either an EGFP- or an EGFP-Gmip-expressing vector (pEGFP-N1 or pEGFP-N1-Gmip) using an Amaxa Nucleofector II device (Lonza, Geneva, Switzerland). The transfected cells were suspended in RPMI-1640 medium (Invitrogen) and re-aggregated, and the aggregates were then cut into blocks (150–200 μm in diameter), embedded in 60% Matrigel/L-15 and cultured for 2.5 days. Live imaging of the cells migrating from the blocks was performed at 2–2.5 days in vitro . Time-lapse images were automatically captured at 6-min intervals for 6–12 h using an LSM710 laser-scanning confocal microscope (Carl Zeiss) and a C-Apochromat × 40/1.20 water objective lens, as specified. FRET-based imaging of active RhoA The FRET probe for RhoA (pRaichu-1298x; ref. 59 ) was kindly provided by Dr Michiyuki Matsuda, Kyoto University. FRET-based imaging for RhoA activity in KD cells was performed essentially as described previously [31] . The three-dimensional Matrigel culture used for the time-lapse imaging of migrating new neurons was performed as described in the previous section. The constructs used in this study were as follows: pRaichu-1,298x (RhoA biosensor), control or Gmip KD vector (pCAGGS-DsRed-miR-LacZ or pCAGGS-DsRed-miR-Gmip) and KD-resistant form Gmip expression vector (ptdTomato, ptdTomato-Gmip* or ptdTomato-GmipΔGAP*). Images for FRET were captured using a Zeiss LSM710 laser-scanning confocal microscope and a C-Apochromat × 40/1.20 water objective lens, as specified. Time-lapse images were automatically captured at 10-min intervals for 6–12 h. The CFP channel was excited using a 458 nm argon line. The two emission channels were split using a 510-nm dichroic mirror and a 460–500 nm band-pass filter for CFP and a 520–560 nm long-pass filter for yellow fluorescent protein (YFP) (Chroma). The confocal aperture size and image size were set at 600 μm and 512 × 512 pixels with a zoom factor of 1.0, respectively. In the time-lapse imaging experiment, all of the new neurons that expressed the RhoA biosensor were continuously migrating for >1 h were analysed. In the KD and rescue experiments, all the new neurons in which expressions of the RhoA biosensor, KD sequence and KD-resistant Gmip mutants were confirmed using MetaMorph software (Molecular Devices, Sunnyvale, CA) were analysed. The ratio image of FRET/CFP was created with MetaMorph software and used to represent the FRET ratio, which was calculated by the following equation: FRET ratio=intensity of FRET/CFP. To examine the distribution of active RhoA in new neurons, the FRET ratio was measured by line scan along the somatic long axis when the swelling formed. The whole cell body was segmented into six regions, as shown in Fig. 4a , and the average FRET ratio of each region was calculated and normalized by dividing by the value of the distal shaft of the leading process. RhoA activity at the proximal leading process was analysed using freehand region of interest (ROI) and region measurement function of MetaMorph software. Statistical analysis All data are shown as means±s.e.m. Comparison of two groups was analysed using an unpaired, two-tailed t -test ( Figs 2o , 3c,e,g–i and 5b,d ; Supplemetary Figs 5, 6c and 8 ; and Supplementary Table 1 ). Multiple group comparisons were performed by one-way ANOVA (Friedman test with Dunn’s test or Kruskal–Wallis test; Figs 2c,g,l , 4b,d and 5f ). A value of P <0.05 was considered as statistically significant. The analyses were performed by Prism 5.0 software (GraphPad, La Jolla, CA). How to cite this article: Ota, H. et al. Speed control for neuronal migration in the postnatal brain by Gmip-mediated local inactivation of RhoA. Nat. Commun. 5:4532 doi: 10.1038/ncomms5532 (2014).